Probing the electron states and metal-insulator transition mechanisms in molybdenum disulphide vertical heterostructures The metal-insulator transition is one of the remarkable electrical properties of atomically thin molybdenum disulphide. Although the theory of electron–electron interactions has been used in modelling the metal-insulator transition in molybdenum disulphide, the underlying mechanism and detailed transition process still remain largely unexplored. Here we demonstrate that the vertical metal-insulator-semiconductor heterostructures built from atomically thin molybdenum disulphide are ideal capacitor structures for probing the electron states. The vertical configuration offers the added advantage of eliminating the influence of large impedance at the band tails and allows the observation of fully excited electron states near the surface of molybdenum disulphide over a wide excitation frequency and temperature range. By combining capacitance and transport measurements, we have observed a percolation-type metal-insulator transition, driven by density inhomogeneities of electron states, in monolayer and multilayer molybdenum disulphide. In addition, the valence band of thin molybdenum disulphide layers and their intrinsic properties are accessed. Molybdenum disulphide (MoS 2 ), an n -type semiconductor [1] , [2] , [3] , [4] , [5] , [6] , [7] , [8] , [9] , [10] , [11] , [12] , [13] , [14] , [15] , [16] , shows novel properties such as superconductivity [6] , controllable valley polarization [17] , [18] and metal-insulator transition [3] , [4] , [5] , [6] (MIT). In MoS 2 field-effect transistors (FETs), gate-induced charge carriers transport in a thin layer near the surface of MoS 2 and are vulnerable to charge impurities and different types of disorder [2] , [3] , [12] , [14] , [19] , [20] . The presence of a high- κ dielectric material [3] to monolayer MoS 2 can effectively screen charge impurities and allow the observation of MIT. Based on recent transport measurements [3] , the phase transition behaviour of monolayer MoS 2 has been attributed to transition from an insulating phase, in which disorder suppresses the electronic interactions, to a metallic phase in which strong coulomb interactions occur. However, the underlying physical mechanism and detailed MIT process need to be further clarified. Different from the studies on transport properties of MoS 2 , the capacitance spectroscopy [14] recently applied to the characterization of MoS 2 FET structures has been demonstrated as one of the most convenient and powerful method for studying the electron states in MoS 2 at room temperature. At low temperatures, however, the information obtained by this technique is limited due to the large impedance near the band edge of MoS 2 . Different from that in graphene quantum capacitors [21] , [22] , [23] , [24] , [25] , [26] , [27] , the slow charge-carrier mobility in MoS 2 capacitors often leads to incompletely charged states, mainly due to the localization near the band edge. The incompletely charged capacitance confuses the effect of charge traps. In the following, we show an approach to address these problems by introducing a MoS 2 -based vertical metal-insulator-semiconductor-metal (MIS-M) heterostructure suitable for probing electron states using capacitance measurements. Unlike conventional FET structures [14] , our approach eliminates the impedance effects and can directly access the intrinsic characteristics of thin-layer MoS 2 over a wide frequency (100 Hz–1 MHz) and temperature range (2–300 K). By combining capacitance and transport measurements, we show that the MIT observed in monolayer and multilayer MoS 2 is consistent with the physical picture of a percolation [28] , [29] , [30] , [31] , [32] , [33] , [34] , [35] transition model. The results of our investigation on the mechanisms of MIT and other intrinsic characteristics, such as thickness-dependent screening abilities and fast relaxation of hole carriers at the valence band, provide useful information much needed for improving the performance of the FET devices based on MoS 2 monolayers and multilayers. 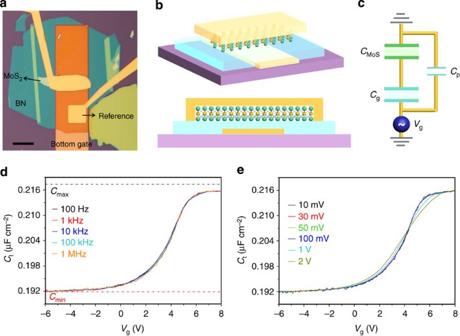Figure 1: The optical and schematic images of the MoS2MIS-M heterostructures. (a,b) The MoS2flakes are fully covered by a top Ti/Au electrode. The square top electrode inais the reference capacitor. Scale bar, 10 μm. (c) The equivalent circuit of the MoS2capacitance devices. Total capacitanceCtmeasured from a 5.9-nm-thick MoS2at 2 K at different frequencies (d) and excitation voltages (e), respectively. The measured capacitance in vertical heterostructures is almost independent of excitation frequencies, which differs greatly from that obtained in conventional FET structures (Supplementary Fig. 4). The excitation voltage used fordis 50 mV and the frequency used foreis 100 kHz. MoS 2 vertical heterostructural capacitance devices Figure 1a,b illustrates our specially designed MIS-M capacitor device, fabricated by transferring [23] , [36] exfoliated flakes of MoS 2 and hexagonal boron nitride (BN) on a Si substrate coated with a SiO 2 thin layer (300 nm). Exfoliated natural crystals of monolayer or multilayer MoS 2 were first transferred onto a BN sheet, serving as an ultra-smooth and disorder-free gate dielectric [37] . A Ti/Au (10 nm/20 nm) local gate sits underneath the BN sheet. The critical step in achieving MIS-M structure is to have the MoS 2 sheet fully covered by a top electrode (Ti/Au: 10 nm/50 nm). The equivalent circuit of this device geometry is shown in Fig. 1c . The measured capacitance C t is the total capacitance contributed by two capacitors originating from MoS 2 ( C MoS ) and the geometric capacitor ( C g ) in serial connection, plus the residual capacitance C p in parallel connection. C t , shown below, is the capacitance wiping off C p (see detailed analysis in Supplementary Figs 1–3 and Supplementary Note 1 and 2 ). Therefore, . With fully covered top electrodes, carriers can respond vertically instead of moving in the plane of MoS 2 . This unique structure directly avoids the huge lateral resistance R of MoS 2 near the band edge. As a result, the measured C t (of a 5.9-nm-thick MoS 2 ) at 2 K ( Fig. 1d ) is almost independent of excitation frequencies f , which differs greatly from that obtained in conventional FET structure devices [7] , [14] . In capacitance measurement of conventional FET structures, lateral resistance R must be considered when R ~1/(2 πfC t ). This is confirmed by our MoS 2 capacitance devices with partially covered top electrodes, which show significant frequency-dependent and temperature-dependent characteristics ( Supplementary Fig. 4 and Supplementary Note 3 ). We also achieved good Ohmic contacts between the top Ti/Au electrode and MoS 2 in our devices, as evidenced by the capacitance measurements at different excitation voltages ( Fig. 1e ). Note that the capacitance measured at large excitation voltages (for example, at 2 V) shows deviation due to the averaging effect. Figure 1: The optical and schematic images of the MoS 2 MIS-M heterostructures. ( a , b ) The MoS 2 flakes are fully covered by a top Ti/Au electrode. The square top electrode in a is the reference capacitor. Scale bar, 10 μm. ( c ) The equivalent circuit of the MoS 2 capacitance devices. Total capacitance C t measured from a 5.9-nm-thick MoS 2 at 2 K at different frequencies ( d ) and excitation voltages ( e ), respectively. The measured capacitance in vertical heterostructures is almost independent of excitation frequencies, which differs greatly from that obtained in conventional FET structures ( Supplementary Fig. 4 ). The excitation voltage used for d is 50 mV and the frequency used for e is 100 kHz. Full size image Characterization of the vertical MIS-M structures The interface structure and band diagrams in the MoS 2 -based MIS-M devices are shown schematically in Fig. 4a–d . When the gate voltage V g >0, electrons accumulate at the MoS 2 surface ( Fig. 4b ). The measured capacitance approaches the geometric capacitance C max = C g when V g is sufficiently large, while under negative V g ( Fig. 4c ) electrons are depleted. In this case, the measured capacitance can be described by , where ε MoS and d MoS are the dielectric constant and the thickness of MoS 2 , respectively. This allows us to directly obtain the ε MoS – d MoS relationship of MoS 2 . To accurately extract , the geometric capacitance C g should be carefully treated. Here, an interlayer capacitance C in originated from the interlayer spacing between BN and MoS 2 is included in the calculation of , where C BN is the geometric capacitance of BN. This interlayer capacitance has been applied in previous studies on twisted bilayer graphene [38] , [39] , [40] . Here we estimate this interlayer capacitance C in ~25.3 μF cm −2 with the interlayer dielectric constant ~10 ε 0 and interlayer spacing ~0.35 nm [38] , [40] . The extracted ε MoS with and without including the interlayer capacitance are both shown in Fig. 2 . Figure 4: The percolation transition driven by density inhomogeneity in multilayer MoS 2 . ( a – d ) The schematic band diagrams of metal-BN-MoS 2 -metal structures at flat band ( a ), accumulation region ( b ), depletion region ( c ) and inversion region ( d ). 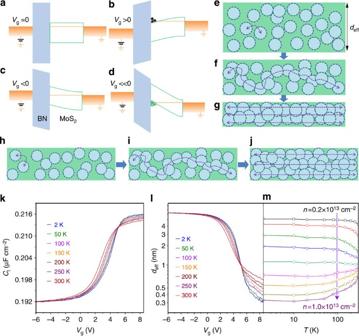Figure 4: The percolation transition driven by density inhomogeneity in multilayer MoS2. (a–d) The schematic band diagrams of metal-BN-MoS2-metal structures at flat band (a), accumulation region (b), depletion region (c) and inversion region (d). (e–j) The schematic images showing the percolation-induced MIT under different effective thicknesses of electron states (e–g) and carrier densities (h–j). The circles denote isolated carrier puddles in MoS2. (k,l) The measured total capacitanceCt(k) and effective thicknessdeff(l) plotted as a function of gate voltageVgfor 2–300 K. The excitation voltage and frequency used are 50 mV and 100 kHz, respectively. (m)deffplotted as a function of temperatures at different carrier densitiesn. ( e – j ) The schematic images showing the percolation-induced MIT under different effective thicknesses of electron states ( e – g ) and carrier densities ( h – j ). The circles denote isolated carrier puddles in MoS 2 . ( k , l ) The measured total capacitance C t ( k ) and effective thickness d eff ( l ) plotted as a function of gate voltage V g for 2–300 K. The excitation voltage and frequency used are 50 mV and 100 kHz, respectively. 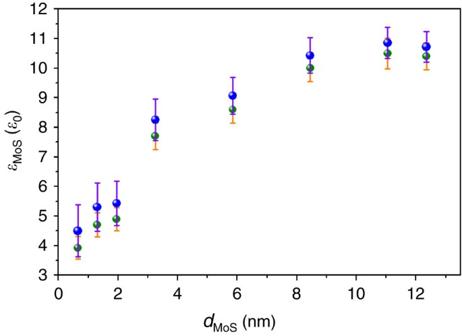( m ) d eff plotted as a function of temperatures at different carrier densities n . Figure 2: Experimental data of the thickness-dependent dielectric constant of MoS2. The dielectric constant of MoS2εMoSwith (blue dots) and without (green dots) including interlayer capacitance is plotted as a function of thicknessdMoS.εMoSincreases from ~4ε0for a monolayer to ~11ε0for bulk MoS2. The errors originate from the measurements of sample sizes, thicknesses of MoS2and BN, and capacitances of MoS2. Full size image Figure 2: Experimental data of the thickness-dependent dielectric constant of MoS 2 . The dielectric constant of MoS 2 ε MoS with (blue dots) and without (green dots) including interlayer capacitance is plotted as a function of thickness d MoS . ε MoS increases from ~4 ε 0 for a monolayer to ~11 ε 0 for bulk MoS 2 . The errors originate from the measurements of sample sizes, thicknesses of MoS 2 and BN, and capacitances of MoS 2 . Full size image As shown in Fig. 2 , ε MoS has been found to increase from ~4 ε 0 for a monolayer to ~11 ε 0 for bulk MoS 2 . This is in excellent agreement with theoretical predictions [41] , [42] . The small ε MoS in monolayer MoS 2 suggests poor dielectric screening of Coulomb interactions, indicating that strong electron–electron interactions could be achieved in clean monolayer MoS 2 . The largely increased mobility observed in monolayer MoS 2 placed in a high- κ dielectric environment [2] , [3] , [43] probably benefits from its small ε MoS . In fact, the decrease in the optical phonon mode observed by a Raman spectroscopy study of few-layer and bulk MoS 2 (ref. 44 ) is also due to the strong dielectric screening effects. The valence band of multilayer MoS 2 is also accessed by detecting the inversion layer of holes using low excitation frequencies at sufficiently high temperatures ( Fig. 3a,b ). However, the inversion layer is invisible when using high frequencies at low temperatures ( T <100 K). This is due to the presence of the Schottky barrier between the Ti/Au contact and the valence band [7] . Holes must form through thermal excitations or minute current leakage into the contacts. This process often requires a long time from ~ms to seconds. In the 12-nm-thick MoS 2 capacitance device, the majority of hole carriers have been relaxed around 20 kHz at 300 K, as confirmed by the phase information of the device, which is defined by Θ=arctan( G /2 πfC t ), where G is the conductance. As shown in Fig. 3c , the phase peaks appear at ~20 kHz for different negative gate bias voltages, indicating that the relaxation time of holes in the 12-nm-thick MoS 2 device is around 50 μs. For the capacitance samples contacted by Cr/Au top electrodes (Cr has a larger work function (~4.5 eV) than that of Ti (~4.3 eV)), a short relaxation time (~5 μs) for holes has also been achieved at 300 K ( Supplementary Fig. 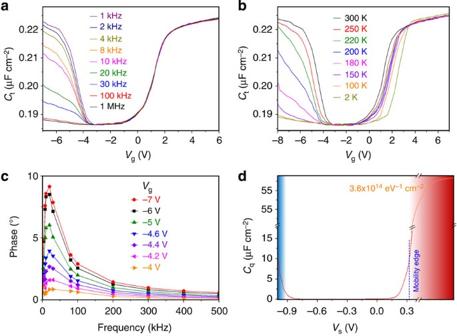5 and Supplementary Note 4 ). Figure 3: The valence band of multilayer MoS2accessed by capacitance measurement. (a)Ctmeasured at 300 K for different excitation frequencies. (b)Ctmeasured at 1 kHz for different temperatures. (c) Phase information plotted as a function of excitation frequencies at 300 K for differentVg. The phase peak around 20 kHz yields a relaxation time of hole carriers at 50 μs. (d) The quantum capacitanceCqof MoS2plotted as a function of surface potentialVsat 300 K, which yields a band gap width of around 1.14 eV. The excitation voltage used is 100 mV. The dashed line above breaks schematically shows the expected quantum capacitance at higher Fermi energies. Figure 3: The valence band of multilayer MoS 2 accessed by capacitance measurement. ( a ) C t measured at 300 K for different excitation frequencies. ( b ) C t measured at 1 kHz for different temperatures. ( c ) Phase information plotted as a function of excitation frequencies at 300 K for different V g . The phase peak around 20 kHz yields a relaxation time of hole carriers at 50 μs. ( d ) The quantum capacitance C q of MoS 2 plotted as a function of surface potential V s at 300 K, which yields a band gap width of around 1.14 eV. The excitation voltage used is 100 mV. The dashed line above breaks schematically shows the expected quantum capacitance at higher Fermi energies. Full size image By applying the Poisson equation to model the vertical heterostructures in a quasi-quantitative manner ( Supplementary Note 5 ), we correlated the quantum capacitance of MoS 2 C q with the surface potential V s in our capacitance devices. V s is extracted based on the charge conservation relation . To accurately extract C q , the interlayer capacitance between BN and MoS 2 C in is included. Owing to the finite thickness of MoS 2 (<15 nm) and the vertical configuration of the capacitance device, the MoS 2 capacitance in vertical structure is a non-zero value C s0 inside the bandgap ( Supplementary Figs 6 and 7 ). The quantum capacitance of MoS 2 C q can be described by C q = C MoS − C s0 ( Supplementary Fig. 8 ). The C q – V s relation is shown in Fig. 3d , yielding a band gap around 1.14 eV, which is close to the reported value of 1.2 eV [45] . The quantum capacitance of monolayer MoS 2 is shown in Supplementary Fig. 9 , which shows a smaller value compared with that in multilayer MoS 2 ( Supplementary Note 6 ). As our measurements are performed near the band edge of MoS 2 and a large amount of disorders are present in MoS 2 , the quantum capacitance is not saturated to the predicted value 57.6 μF cm −2 (corresponding to a density of states ~3.6 × 10 14 eV −1 cm −2 (refs 14 , 46 )) beyond the mobility edge. The dashed line above breaks in Fig. 3d schematically shows the expected quantum capacitance at higher Fermi energies. Percolation-induced MIT in monolayer and multilayer MoS 2 Similar to the MIT observed in transport measurements [3] , [4] , [5] , [6] , the capacitance data of the 5.9-nm-thick MoS 2 device measured at different temperatures ( Fig. 4m ) show an interesting transition with a well-defined cross-over point (at V g =5 V and corresponding to a carrier density n ~6.8 × 10 12 cm −2 , obtained from n = C g ( V g − V s − V T )/ e , where V T ~−1 V is the threshold voltage). When V g <5 V C t decreases with decreasing temperature, whereas at V g >5 V the temperature dependence of C t is reversed. The observed cross-over point in capacitance measurements is indeed related to the MIT as its value (~6.8 × 10 12 cm −2 ) is consistent with that measured by transport (ref. 6 and Fig. 6 ). More evidence is provided by capacitance measurements of monolayer MoS 2 samples ( Fig. 5a ). In monolayer MoS 2 , the intersections of the capacitance curves showed obvious temperature-dependent characteristics. At temperatures below 100 K, we observed that the cross-over point was stabilized roughly at n ~1.2 × 10 13 cm −2 , consistent with the transport results measured in monolayer MoS 2 (ref. 3 ) with an MIT at n ~1 × 10 13 cm −2 . Bilayer and trilayer MoS 2 samples displayed similar transition phenomena with cross-over points around n ~8.6 × 10 12 cm −2 ( Fig. 5b ). Figure 6: Transport results showing the percolation transition in multilayer and monolayer MoS 2 . 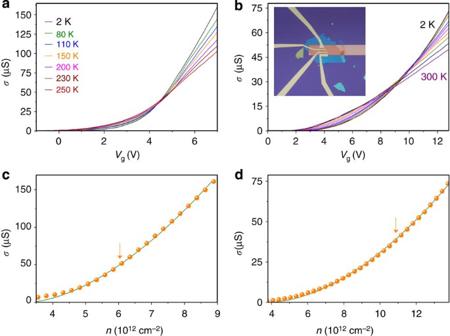Figure 6: Transport results showing the percolation transition in multilayer and monolayer MoS2. (a,b) The MITs are clearly shown byσmeasurements of a multilayer (a) and monolayer (b) MoS2for different temperatures. The inset inbshows the optical image of a monolayer MoS2device. (c,d) The fitting of experimentalσ(orange dots) of multilayer (c) and monolayer (d) MoS2according to the percolation conductivityσ=A(n−nc)δ(green lines). The arrows denote the positions of MITs. ( a , b ) The MITs are clearly shown by σ measurements of a multilayer ( a ) and monolayer ( b ) MoS 2 for different temperatures. The inset in b shows the optical image of a monolayer MoS 2 device. ( c , d ) The fitting of experimental σ (orange dots) of multilayer ( c ) and monolayer ( d ) MoS 2 according to the percolation conductivity σ = A ( n − n c ) δ (green lines). 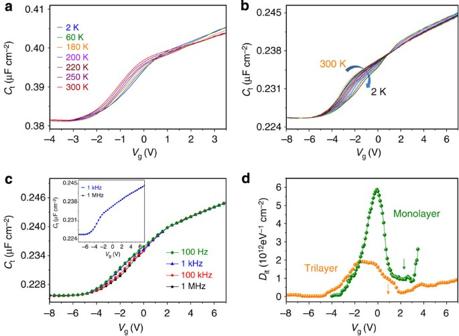The arrows denote the positions of MITs. Figure 5: The percolation transition and charge traps in monolayer and trilayer MoS2. (a)Ctof a monolayer MoS2measured at an excitation frequency 1 kHz and excitation voltage 50 mV for different temperatures. (b)Ctof a trilayer MoS2measured at an excitation frequency 100 kHz. (c)Ctof a trilayer MoS2measured for different excitation frequencies at 2 K, indicating that the charge traps are excited at low frequencies. The inset showsCtmeasured at 300 K. (d) The charge-trap densitiesDitas a function ofVgcalculated for the monolayer and trilayer MoS2samples. The arrows denote the transition points. Full size image Figure 5: The percolation transition and charge traps in monolayer and trilayer MoS 2 . ( a ) C t of a monolayer MoS 2 measured at an excitation frequency 1 kHz and excitation voltage 50 mV for different temperatures. ( b ) C t of a trilayer MoS 2 measured at an excitation frequency 100 kHz. ( c ) C t of a trilayer MoS 2 measured for different excitation frequencies at 2 K, indicating that the charge traps are excited at low frequencies. The inset shows C t measured at 300 K. ( d ) The charge-trap densities D it as a function of V g calculated for the monolayer and trilayer MoS 2 samples. The arrows denote the transition points. Full size image The electronic transport of MoS 2 suffers from charge impurities [2] , [3] and short-range disorders [12] , [14] , [19] , [20] , such as ripples, dislocation and sulphur vacancies. These disorders result in the insulating transport behaviour of MoS 2 in the low carrier-density region, where electrons transport through hopping between localized states ( Fig. 4h ) and can be well described by the variable-range-hopping model [3] , [12] , [20] . In the region where sufficient, large carrier densities are introduced, metal behaviour is observed [3] . Here we propose a percolation-type MIT in MoS 2 , driven by density inhomogeneity of electron states [28] , [29] , [30] , [31] , [32] , [33] , [34] , [35] that describes the systems in which charge carriers are transported through percolating conductive channels in the disorder landscapes due to the poor screening effect at low carrier densities. When carrier density is low enough, conductive paths are efficiently blocked and MIT occurs. MoS 2 has been proven to be such a disordered system, with impurity concentration ranging from 10 11 to 10 13 cm −2 , especially for monolayer MoS 2 , which is more vulnerable to ripples and charge impurities [2] , [3] , [12] , [14] , [19] , [20] . Thus, the MIT in MoS 2 is in line with the percolation transition theory in which disorder plays an important role. Moreover, our capacitance and transport data, shown below, provide further evidences to this effect. The evolution of concentration and effective thickness of electron states probed by capacitance measurements can explain the observed MIT in transport measurements fairly well and provide details of the percolation transition process. The percolation transition phenomenon is illustrated in Fig. 4h–j . With increasing carrier densities n (by increasing gate voltage), the localized electron states begin to percolate with each other till a conductive channel occurs at a critical density ( Fig. 4i ). Further increasing carrier densities will lead to sufficient conductive channels spanning the entire system and result in metal-like transport behaviours ( Fig. 4j ). On the other hand, at the same carrier density, the effective thickness d eff = ε MoS / C MoS of electron states confined in the surface of MoS 2 can be tuned by varying temperatures ( Fig. 4l ). Smaller d eff can also be achieved at higher gate voltages where large amounts of surface charges are induced (supported by theoretical calculations in the Supplementary Note 5 ). As illustrated in Fig. 4e–g (assuming n remains unchanged), more conductive channels are formed at a smaller d eff . The MIT should occur when d eff is sufficiently small. The capacitance data of our samples ( Fig. 4l,m ) are similar to those obtained from transport measurements in multilayer MoS 2 (showing an MIT at n =6.7 × 10 12 cm −2 ) (ref. 6 ). When n <6.8 × 10 12 cm −2 , d eff decreases with increasing temperatures. Hence, the conductivity should increase as the temperature increases. In contrast, when n >6.8 × 10 12 cm −2 , the increase of d eff would lead to decreasing conductivity as the temperature increases. Furthermore, the increasing n and decreasing d eff would also enhance the screening of disorders and electron states, and thus lead to increasing conductivity, while lowering the Coulomb interaction strength. It is noticed that the effective channel thickness is only applicable to multilayer MoS 2 , as monolayer MoS 2 is a truly 2D system. The percolation transition in monolayer MoS 2 mainly results from the tuning of concentration of electron states at different gate voltages. An alternative explanation on the transition is based on the quantum capacitance of MoS 2 , which is closely related to the carrier density and the effective channel thickness. A larger quantum capacitance suggests a larger density of states or a smaller effective channel thickness. Therefore, the observed gate-tuned transition from insulating to metallic region is the direct consequence of the increase of quantum capacitance with increasing gate voltages (as shown in Fig. 3d ). The percolation transition also suggests an increasing transition density at the cross-over point with increasing impurity concentration [30] , [31] , [32] . In our MoS 2 samples, the transition density was in the range 10 12 –10 13 cm −2 due to the presence of large amounts of impurities. Moreover, the transition density in monolayer MoS 2 (~1 × 10 13 cm −2 ) was larger than that observed in multilayer MoS 2 (~6 × 10 12 cm −2 ), which agreed with the prediction of percolation theory as monolayer MoS 2 was more vulnerable to disorders. This was further evidenced by extracting charge trap densities, D it , of MoS 2 from capacitance measurements (a trilayer sample shown in Fig. 5c ). The presence of impurities or disorder may cause charge-trapping effects in MoS 2 capacitance devices, particularly at low temperatures. The charge traps can be fully excited only at relatively low frequencies (for example, 100 Hz). The density of the charge traps can then be estimated by measuring the difference in capacitance at low and high frequencies, that is, D it =( C MoS ( low _ f )– C MoS ( high _ f ))/ e . The trap densities in our monolayer and trilayer MoS 2 samples were in the order of 10 12 eV −1 cm −2 ( Fig. 5d ). The trap densities in monolayer MoS 2 were apparently large, suggesting that monolayer MoS 2 is more sensitive to disorder. In fact, the trap densities in our samples were underestimated because of the limitation of the excitation frequency ranges. At relatively high temperatures (inset of Fig. 5c ), the charge traps were easily excited and the capacitances measured at low and high frequency show no difference. The percolation-induced MIT in MoS 2 is further supported by transport data at low temperatures. The MITs of multilayer ( Fig. 6a ) and monolayer ( Fig. 6b ) MoS 2 are clearly shown by the conductivity σ , at different temperatures, similar to previous reports [3] , [4] , [5] , [6] . The MIT occurs at n ~6 × 10 12 cm −2 for multilayer MoS 2 and n ~1.1 × 10 12 cm −2 for monolayer MoS 2 , consistent with the capacitance data. The mobilities of the monolayer and multilayer MoS 2 samples measured at 2 K are around 90 and 250 cm 2 V −1 s −1 , respectively ( Supplementary Fig. 10 and Supplementary Note 7 ). To gain further insight into the transition behaviour, we applied the percolation model of conductivity [31] , [32] , [35] near the percolation threshold density n c , which is described by where A is a constant of proportionality and δ is the percolation exponent. Below the threshold density n c , the 2D electron gas broke up into isolated puddles of carriers, with no conducting channels crossing the whole sample. The conductivity showed insulating behaviour and eventually vanished at T =0 K. In 2D systems, δ is expected to be 4/3 and a cross-over point (~ e 2 / h ) above the percolation threshold density is suggested at finite temperatures [30] , [31] . Based on the percolation model, we fit our experimental data of multilayer ( Fig. 6c ) and monolayer ( Fig. 6d ) MoS 2 samples at 2 K. The experimental results show excellent agreement with theoretical predictions near the transition point. The extracted parameters are δ ~1.7 and n c ~3.2 × 10 12 cm −2 in multilayer MoS 2 and δ ~1.8 and n c ~3.8 × 10 12 cm −2 in monolayer MoS 2 . The obtained percolation exponents are consistent with experimental values δ =1.4–1.7 found in other 2D systems, such as GaAs/AlGaAs heterostructures [31] , [32] . The obtained percolation threshold density n c is lower than the value of MIT cross-over point (mobility edge) because of thermal activation of localized electron states. n c would approach the mobility edge when temperature is sufficiently low. The percolation transition model can be applied only near the transition point at low temperatures. In the metallic region with higher carrier densities, the conductivity would show a linear increase with gate voltages where the conductivity is mainly limited by the linearly screened charge impurity scattering [31] . The slight deviation between experimental data and fitting curves at low carrier densities is due to enhanced hopping conductivity and quantum tunnelling at finite temperatures. One alternative scenario besides the percolation transition model is the phase transition theory for a metallic phase (stabilized by e – e interactions) and an insulating phase (disorder prevails over e – e interactions), which are separated by a quantum critical point [3] , [47] . This theory shows the existence of the quantum critical point where the density of states of the underlying collective modes is divergent at the transition point. The transport data obtained from MoS 2 cannot provide more information for distinguishing these divergent collective modes. In contrast, the capacitance measurement is able to probe the global behaviour of these divergent collective modes, which would lead to a divergent quantum capacitance at the transition point [22] , [25] , [47] . In our capacitance experiments, however, the divergent quantum capacitance was not observed around the transition point. The capacitance data seems to be more inclined to the density inhomogeneity induced by disorder, which dominates the properties at the MIT transition point, as the Coulomb interactions of electrons could be suppressed by a large amount of disorder existing in MoS 2 . Based on our transport and capacitance data, the percolation transition model is more consistent with the MIT phenomena in MoS 2 . The vertical MIS heterostructures built from atomically thin MoS 2 are ideal capacitor structures for probing the electron states and intrinsic properties of MoS 2 . According to the analyses of experimental data obtained by electrical transport measurement and capacitance spectroscopy, we believe that the percolation-type MIT (driven by density inhomogeneities of electron states) is the dominating mechanism of the MIT in both monolayer and multilayer MoS 2 . The vertical heterostructures offer the added advantages of eliminating the influence of large impedance at the band tails and accessing intrinsic characteristics such as thickness-dependence dielectric constant and band gap variation in atomically thin MoS 2 . The present study also provides a new approach to characterizing the intrinsic properties of other atomically thin-layered materials and interface states of heterostructures built from 2D materials. Sample preparation Monolayer and multilayer MoS 2 flakes were exfoliated from MoS 2 crystals (from 2D semiconductors) by the micromechanical cleavage technique. MoS 2 and BN flakes were placed on the surface of a glass slide coated with Polydimethylsiloxane/Methyl methacrylate as described for graphene-BN device fabrication [36] . Next, these thin flakes were transferred onto a local Ti/Au (10 nm/20 nm) gate. The top electrodes were patterned using standard electron-beam lithography. Two types of top electrodes, Ti/Au (10 nm/50 nm) and Cr/Au (2 nm/50 nm), were fabricated through electron-beam evaporation. The dielectric constant of the BN sheet is measured by calibrating an internal reference capacitor that sits near the MoS 2 capacitance device ( Fig. 1a ). The thicknesses of MoS 2 and BN flakes were measured by an atomic force microscope (Veeco-Innova). Capacitance and transport measurements Capacitance measurements were carried out using an HP Precision 4284A LCR Meter with a sensitivity of ~0.1 fF in a cryogenic system (2–300 K). All wires in the measurement circuits were shielded and the p-Si substrates were also grounded to minimize residual capacitance. The residual capacitance in the measurement setup is at the order of 1 fF (see Supplementary Fig. 3 ). Transport measurements were performed in the same cryogenic system using lock-in techniques. How to cite this article: Chen, X. et al . Probing the electron states and metal-insulator transition mechanisms in molybdenum disulphide vertical heterostructures. Nat. Commun. 6:6088 doi: 10.1038/ncomms7088 (2015).